Synthetic RNA devices to expedite the evolution of metabolite-producing microbes An extension of directed evolution strategies to genome-wide variations increases the chance of obtaining metabolite-overproducing microbes. However, a general high-throughput screening platform for selecting improved strains remains out of reach. Here, to expedite the evolution of metabolite-producing microbes, we utilize synthetic RNA devices comprising a riboswitch and a selection module that specifically sense inconspicuous metabolites. Using L -lysine-producing Escherichia coli as a model system, we demonstrated that this RNA device could enrich pathway-optimized strains to up to 75% of the total population after four rounds of enrichment cycles. Furthermore, the potential applicability of this device was examined by successfully extending its application to the case of L -tryptophan. When used in conjunction with combinatorial mutagenesis for metabolite overproduction, our synthetic RNA device should facilitate strain improvement. Microbial engineering for the production of chemicals relies on the rational design of metabolic pathways so as to redirect the metabolic flux towards a particular metabolite [1] , [2] , [3] , [4] . Improving product yields or pathway efficiencies, however, requires optimization of various metabolic pathways in the cellular metabolism—a difficult task using rational approaches [5] . Advances in generating diverse cellular phenotypes have made it possible to achieve a desired phenotype through directed evolution [6] , [7] , [8] , [9] . Nevertheless, because a majority of target products of interest are not associated with a conspicuous phenotype, the improved strains are beyond the reach of a general screening tool and cannot be readily obtained [10] . These limitations argue for the development of a novel screening device that satisfies the following three conditions: One is ability to sensitively detect the target products, another is capacity for high-throughput screening, and the other is universal applicability to inconspicuous products. In nature, RNA segments act to sense cellular information and, based on that information, regulate genetic expression at the levels of transcription, translation and RNA degradation [11] . Among such RNA segments, riboswitches—noncoding cis -regulatory elements found in the 5′-untranslated regions of mRNAs—typically sense intracellular metabolites through aptamer domains, which bind these metabolites and undergo a metabolite-induced conformational change that converts the metabolic signal into a change in the expression of downstream genes [12] . RNA aptamers that bind to target molecules with high selectivity and sensitivity can be readily selected in vitro through systematic evolution of ligands by exponential enrichment [13] . Synthetic riboswitches that actually work in vivo can be generated from these in vitro -selected aptamers and can also be functionally manipulated using various high-throughput screening methods [14] , [15] , [16] . In this study, we anticipated that a genetic device comprising riboswitch-based RNA sensors could be used to monitor the alteration of cellular phenotypes caused by changes in the intracellular concentration of a specific metabolite in precisely the same manner as the corresponding riboswitches function in nature [17] , [18] and to optimize cellular metabolisms for improved yield and productivity of the target molecules. We demonstrated that this RNA device could enrich pathway-optimized strains by specifically sensing the L -lysine in E. coli . Furthermore, the applicability of this synthetic device was examined by successfully extending its application to the case of L -tryptophan. The potential of such a device to specifically sense various inconspicuous target molecules offers the promise of the possible extension as a screening method for efficient strain improvement [19] . A synthetic RNA device as a platform for strain improvement To expedite the evolution of metabolite-producing microbes, we sought to utilize a synthetic RNA device (called a Riboselector) comprising two modules: one is a riboswitch module for sensing the intracellular concentration of a specific metabolite and actuating the regulation of gene expression based on metabolite signals, and the other is a selection module enabling high-throughput screening ( Fig. 1a ). Although this genetic device has been used for screening the genetic switches [16] or probing the genetic pathways [18] , we anticipated that this device might also be utilized as a platform for efficient strain improvement in the way that it can convert the cellular metabolic information into a conspicuous phenotype, such as survival under selection pressure. 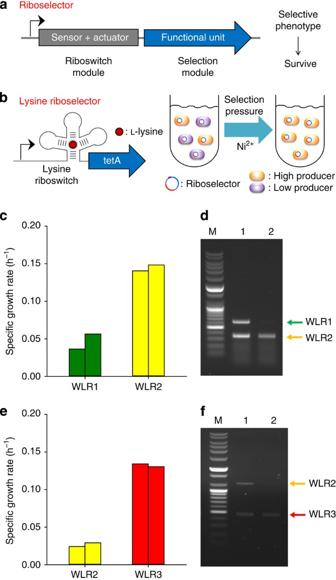Figure 1: A synthetic RNA device (Riboselector) and its implementation forL-lysine production. (a) A Riboselector is comprised of two modules: a riboswitch and a selection module. (b) The Lysine Riboselector consisting of a lysine riboswitch fromlysCofE. coliand the selection markertetAenriches the high lysine producer in the presence of NiCl2. (c–f) The relatively high lysine producer grew more rapidly and was enriched under selection pressure following introduction of the Lysine Riboselector. Theyaxis in (c) and (e) represents the specific growth rate (h−1), and the experiments were replicated twice. Lanes M, 1 and 2 in (d) and (f) represent the molecular marker, mixed culture of strains without the Lysine Riboselector, and mixed culture of strains with the Lysine Riboselector, respectively. Target regions for amplification and expected sizes were as follows: (d)lysC(605 bps for WLR1 and 343 bps for WLR2), (f)iclR(1,173 bps for WLR2, 408 bps for WLR3). Selection conditions were as follows: (c,d) 21 μM NiCl2in M9 media, and (e,f) 240 μM NiCl2in complemented M9 media. Figure 1: A synthetic RNA device (Riboselector) and its implementation for L -lysine production. ( a ) A Riboselector is comprised of two modules: a riboswitch and a selection module. ( b ) The Lysine Riboselector consisting of a lysine riboswitch from lysC of E. coli and the selection marker tetA enriches the high lysine producer in the presence of NiCl 2 . ( c – f ) The relatively high lysine producer grew more rapidly and was enriched under selection pressure following introduction of the Lysine Riboselector. The y axis in ( c ) and ( e ) represents the specific growth rate (h −1 ), and the experiments were replicated twice. Lanes M, 1 and 2 in ( d ) and ( f ) represent the molecular marker, mixed culture of strains without the Lysine Riboselector, and mixed culture of strains with the Lysine Riboselector, respectively. Target regions for amplification and expected sizes were as follows: ( d ) lysC (605 bps for WLR1 and 343 bps for WLR2), ( f ) iclR (1,173 bps for WLR2, 408 bps for WLR3). Selection conditions were as follows: ( c , d ) 21 μM NiCl 2 in M9 media, and ( e , f ) 240 μM NiCl 2 in complemented M9 media. Full size image To demonstrate proof of principle, we chose L -lysine, whose naturally existing riboswitches have been extensively studied and characterized, as a target metabolite [20] , [21] . To construct strains with different intracellular concentrations of lysine, we chose lysC , an aspartokinase isozyme, as a target to modulate the metabolic flux from oxaloacetate to lysine. In a previous study, a lysC knockout strain showed a lysine starvation response, reflecting the fact that the other two isozymes are regulated by methionine and threonine [22] , [23] . We found that the leader sequences of E. coli lysC positioned upstream of the green fluorescent protein reporter gene ( sgfp ) could serve as a genetic control element to repress the expression of the downstream gene in a manner that depended on the intracellular lysine concentration [21] (WL0 and WL1; Supplementary Figs S1 and S2 ). To construct a ‘Lysine Riboselector’, we combined this leader region of E. coli lysC with the selection marker tetA encoding a tetracycline/H + antiporter ( Fig. 1b ). Although this lysine-responsive genetic device is a repressive type of regulator, the dual-selection modes of TetA enable cells that accumulate lysine in the cytoplasm to survive in the presence of toxic metal salts, such as NiCl 2 [16] . As expected, cellular growth rates were severely affected by the intracellular concentration of lysine only if the functional Lysine Riboselector was implemented ( Supplementary Fig. S3 ). Furthermore, we examined whether it would be possible to modulate the selection cutoff levels of the Lysine Riboselector depending on the intracellular concentration of lysine. To accomplish this, we constructed two other E. coli strains having different intracellular concentrations of lysine. On the basis of the fact that amplification of feedback-resistant lysC showed an increase in lysine production [24] , we constructed WL2 strain to have increased intracellular concentration of lysine compared with WL1. Additional modifications, including overexpression of lysine synthesis pathway and deletion of competing pathways [25] , were made to result in WL3 strain with further increased intracellular concentration of lysine compared with WL2. We confirmed that all the constructed strains showed different intracellular concentrations of lysine as expected ( Supplementary Fig. S1 ). By simply modulating the selection conditions, we were able to observe differences in cellular growth rates between strains ( Fig. 1c ) caused by changes in the expression levels of tetA , which, in turn, reflected the intracellular concentration of lysine in each strain only when the functional Lysine Riboselector was implemented ( Supplementary Figs S4 and S5 ). Moreover, these differences in growth rates enabled us to distinguish between relatively high- and low-lysine producers after several rounds of enrichment culture under selective conditions ( Fig. 1d ). As the binding sensitivity of aptamers towards chemicals, as well as the activation ratio of a riboswitch module, can be customized during the riboselector construction process [15] , [26] , [27] , [28] , the selection cutoff levels could be further modulated according to the physiological conditions of the target strain. Riboselector-driven L -lysine pathway optimization Next, we applied the Lysine Riboselector to select the high lysine producer from among various physiologically diverse microbes. Balancing the flux distributions of anaplerotic and glycolytic pathways around the phosphoenolpyruvate node is critical for enhancing the production of lysine from glucose [29] , [30] . To resolve this problem, we constructed promoter libraries of ppc encoding phosphoenolpyruvate carboxylase, a key anaplerotic enzyme, and attempted to find the optimal expression level of ppc for lysine production by enrichment using the Lysine Riboselector ( Fig. 2a ). The positions for library construction were selected as the consensus hexameric DNA sequences (−10 and −35 boxes) of promoters to yield a large library with a broad range of transcription efficiency (See details in Supplementary Methods ). Selection pressure for the enrichment was set at 90 μM NiCl 2 , which severely hampered the growth of the parental strain only when the Lysine Riboselector was introduced ( Supplementary Fig. S6 ). The plasmid library was transformed into WLR4 harbouring the functional Lysine Riboselector to achieve ppc clones for the screening and also transformed into WLM4 and WLN4 strains as the control experiments. Once the cells are reached to mid-exponential phase, they were diluted in fresh selection medium. However, the library constructed by using the cells harbouring LysRiboMut (WLM4) was failed to grow in selection medium due to the constitutive expression of tetA regardless of the intracellular lysine concentration. After three serial cultures (using ppc clones constructed by using WLR4 and WLN4), which represent each enrichment cycle, enriched plasmids were extracted and retransformed into fresh parental strain to prevent the adaptation of cells to nickel ( Fig. 2b ). After the fourth enrichment cycle, a population analysis of the enriched broth with functional Lysine Riboselector (derived from WLR4) using next-generation sequencing revealed that the top three strains, each with different promoter sequences, accounted for up to 75% of the total population ( Fig. 2c and Supplementary Table S1 ). These three strains (WLRE1, WLRE2 and WLRE3) showed dramatic increases in lysine production compared with the parental strain (WL3), which barely accumulated lysine in the culture broth ( Fig. 2d and Supplementary Fig. S7 ). These results indicate that strains with a ppc expression level optimized for lysine production were successfully enriched. Because the strength of each enriched promoter sequence differed ( Supplementary Fig. S8 ), enriched strains showed slight differences in lysine productivity. As ppc expression levels were further increased, the final lysine titres decreased, an outcome comparable to that obtained in a previous study on threonine, another branch of the aspartate family pathway [31] . 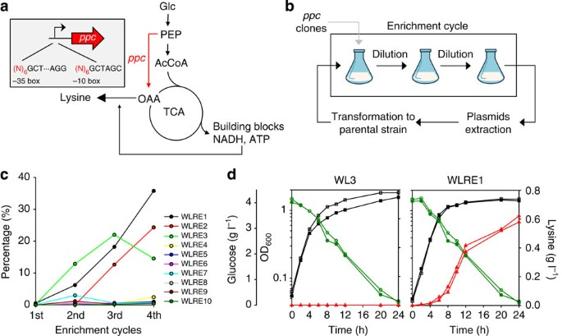Figure 2: Optimization of the lysine metabolic pathway using the Lysine Riboselector. (a) Simplified metabolic pathway leading to lysine production inE. coli. The optimal expression level ofppcwas found by randomizing the −35 and −10 boxes of the promoter (from BBa_J23100) as follows: (N)6GCTAGCTCAGTCCTAGG(N)6GCTAGC, where ‘N’ denotes randomized nucleotides. Glc, glucose; PEP, phosphoenolpyruvate; AcCoA, acetyl-CoA; OAA, oxaloacetate. (b) After three serial cultures ofppcclones, which represent each enrichment cycle, enriched plasmids were extracted and retransformed into fresh parental strain to prevent the adaptation of cells to nickel. (c) Next-generation sequencing was used to examine the promoter region of each variant (enriched by using Lysine Riboselector) for population analysis. Theyaxis represents the percentage of each variant in the total population. Thexaxis represents the enrichment cycle, where each enrichment cycle corresponds to three serial cultures. (d) Physiological comparison between the parental strain (WL3, left panel) and one of the enriched strains (WLRE1, right panel) using LysRibo. The leftyoffset and rightyaxis represent glucose (circles) and lysine (triangles) concentration (g l−1), respectively. The leftyaxis represents optical density (rectangles) at 600 nm in log scale. Thexaxis represents the culture time (h). The experiments were replicated twice. Figure 2: Optimization of the lysine metabolic pathway using the Lysine Riboselector. ( a ) Simplified metabolic pathway leading to lysine production in E. coli . The optimal expression level of ppc was found by randomizing the −35 and −10 boxes of the promoter (from BBa_J23100) as follows: (N) 6 GCTAGCTCAGTCCTAGG(N) 6 GCTAGC, where ‘N’ denotes randomized nucleotides. Glc, glucose; PEP, phosphoenolpyruvate; AcCoA, acetyl-CoA; OAA, oxaloacetate. ( b ) After three serial cultures of ppc clones, which represent each enrichment cycle, enriched plasmids were extracted and retransformed into fresh parental strain to prevent the adaptation of cells to nickel. ( c ) Next-generation sequencing was used to examine the promoter region of each variant (enriched by using Lysine Riboselector) for population analysis. The y axis represents the percentage of each variant in the total population. The x axis represents the enrichment cycle, where each enrichment cycle corresponds to three serial cultures. ( d ) Physiological comparison between the parental strain (WL3, left panel) and one of the enriched strains (WLRE1, right panel) using LysRibo. The left y offset and right y axis represent glucose (circles) and lysine (triangles) concentration (g l −1 ), respectively. The left y axis represents optical density (rectangles) at 600 nm in log scale. The x axis represents the culture time (h). The experiments were replicated twice. Full size image However, when these three selected promoter sequences were introduced into the chromosome (WLCP1, WLCP2 and WLCP3), these strains showed a marginal increase in lysine production or retarded cellular growth compared with the parental strain ( Supplementary Fig. S9 ). Owing to the difference in copy numbers between chromosome-based and plasmid-based expression, expression levels of ppc changed significantly ( Supplementary Fig. S8 ). These results further imply that fine-tuning control of gene expression depending on the expression system is critical for pathway optimization [5] , [32] . In case of the control experiment performed with library constructed by using WLN4 harbouring RiboNULL, no particular promoter sequences are enriched after the fourth enrichment cycle ( Supplementary Fig. S10 ). Furthermore, none of the promoter sequences of them was identical with the previously enriched top three variants using Lysine Riboselector (WLRE1, WLRE2 and WLRE3) ( Supplementary Table S2 ). Among them, we picked three clones (WLNE1, WLNE2 and WLNE3) and examined the lysine production. The lysine productions of them were not significantly increased compared with parental strain ( Supplementary Fig. S11 ), suggesting that the selection process with Lysine Riboselector was specific to lysine overproducers. Taken together, these results indicate that the synthetic RNA device—the Lysine Riboselector—enabled us to easily screen for a high lysine producer from among innumerable potential candidates by specifically sensing the inconspicuous metabolite, L -lysine, without a requirement for additional expensive analytical instruments or methods. Extending the usage of the Riboselector to L -tryptophan Finally, we examined whether the Riboselector has the potential for general application to other inconspicuous metabolites. To demonstrate this, we chose L -tryptophan, whose naturally occurring riboswitch has not yet been discovered, as another inconspicuous target metabolite. As a starting point for the creation of a ‘Tryptophan Riboselector’ [16] , we selected one of the synthetic aptamers specific for L -tryptophan that are already known [33] . The readily obtained Tryptophan Riboselector ( Fig. 3a , see Methods for details) activated tetA-sgfp expression up to 3.5-fold in the presence of 1 mM tryptophan ( Fig. 3b ), an increase that we anticipated would be sufficient to perform as designed in response to changes in physiological conditions [34] . To construct strains with different intracellular concentrations of tryptophan, we chose aroG , a 3-deoxy- D -arabino-heptulosonate-7-phosphate synthase (DS) isozyme, as a target to modulate the metabolic flux towards tryptophan. Because 80% of total DS activity is known to be contributed by aroG [35] , we constructed the WT0 strain by deleting aroG in the chromosome of the W3110 strain. As expected, cellular growth rates of cells harbouring the Tryptophan Riboselector and exposed to selection pressure were severely affected by the intracellular concentrations of tryptophan ( Fig. 3c ). Because this Tryptophan Riboselector was an on-type (unlike the off-type Lysine Riboselector), we could distinguish a relatively high tryptophan producer with several rounds of serial culture in the presence of tetracycline ( Fig. 3d ). In view of the fact that the Lysine Riboselector could be utilized to select a high lysine producer, it is likely that a high tryptophan producer could be easily developed by applying the Tryptophan Riboselector to expedite evolution of tryptophan-producing E. coli [35] . 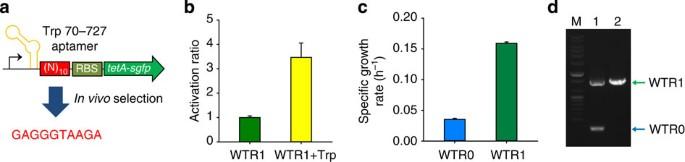Figure 3: Extending the application of the Riboselector toL-tryptophan. (a) A Tryptophan Riboselector was constructed by selecting (N)10sequences capable of functionally connecting the aptamer region with the selection module (tetA-sgfp)in vivo. The selected sequence used was 5′-GAGGGTAAGA-3′. (b) The Tryptophan Riboselector showed 3.5-fold activation with supplementation of 1 mM tryptophan. Theyaxis represents the activation ratio, determined by measuring Riboselector-driven fluorescence. (c,d) The relatively high tryptophan producer grew more rapidly and was enriched under selection pressure (140 μg ml−1tetracycline in M9) following introduction of the Tryptophan Riboselector. Theyaxis increpresents the specific growth rate (h−1). Lanes M, 1 and 2 in (d) represent the molecular marker, mixed culture of strains without the Tryptophan Riboselector and mixed culture of strains with the Tryptophan Riboselector, respectively. The target region for amplification and the expected size were as follows:aroG(1,539 bps for WTR0 and 354 bps for WTR1). The error bars inbandcindicate s.d. of measurements from three independent cultures. Figure 3: Extending the application of the Riboselector to L -tryptophan. ( a ) A Tryptophan Riboselector was constructed by selecting (N) 10 sequences capable of functionally connecting the aptamer region with the selection module ( tetA-sgfp ) in vivo . The selected sequence used was 5′-GAGGGTAAGA-3′. ( b ) The Tryptophan Riboselector showed 3.5-fold activation with supplementation of 1 mM tryptophan. The y axis represents the activation ratio, determined by measuring Riboselector-driven fluorescence. ( c , d ) The relatively high tryptophan producer grew more rapidly and was enriched under selection pressure (140 μg ml −1 tetracycline in M9) following introduction of the Tryptophan Riboselector. The y axis in c represents the specific growth rate (h −1 ). Lanes M, 1 and 2 in ( d ) represent the molecular marker, mixed culture of strains without the Tryptophan Riboselector and mixed culture of strains with the Tryptophan Riboselector, respectively. The target region for amplification and the expected size were as follows: aroG (1,539 bps for WTR0 and 354 bps for WTR1). The error bars in b and c indicate s.d. of measurements from three independent cultures. Full size image Recently, various genetic devices combining the riboswitches with reporter genes have been described to modulate genetic switches, discover the genetic pathway and reprogram cellular behaviours [15] , [16] , [18] , [34] , [36] . However, none of them was directly used for evolving metabolite-producing microbes to increase the yield and the productivity of the target molecules. In this study, we reported how a synthetic RNA device (Riboselector) could be utilized as a platform for efficient strain improvement by successfully demonstrating the optimization of L -lysine-producing pathway in E. coli . Furthermore, we examined the potential applicability of this device by readily developing Tryptophan Riboselector and testing its ability to enrich the relatively high tryptophan producer. The key of utilizing this device for strain improvement relies on how to develop and modulate synthetic riboselectors. In recent decades, an expanding number of riboswitch classes, even those with specificity for the fluoride anion, have been discovered from natural sources [19] , [37] . This indicates that there is a strong possibility of generating synthetic aptamers that selectively bind to numerous chemicals by systematic evolution of ligands by exponential enrichment in which we are interested [13] . Then, synthetic riboselectors based on these in vitro -selected aptamers can be easily constructed by applying any of several high-throughput screening methods as shown in this study [14] , [15] , [16] . Considering a recent advance in engineering RNA devices that enables such devices to quantitatively programme gene expression based on mathematical models [27] , it should be practicable to expand the use of the synthetic RNA devices developed here to various other metabolites. Moreover, by subjecting the synthetic riboselector to a series of in vitro and in vivo selection processes, it is possible to control kinetic components of the device, such as binding affinity and dynamic range, to obtain an RNA device that is functional under the physiological conditions of the parental strain [15] . Once the riboselector is constructed using the aforementioned procedures, iterative strain improvement can be accomplished by simply modulating the selection cutoff levels during the enrichment process ( Fig. 4 ). To engineer robust and genetically stable strains, recently developed techniques for genome-wide alterations of cellular phenotypes might be able to be combined with our strategy to efficiently find optimal strains [6] , [7] , [8] , [9] , [38] , [39] , [40] . Furthermore, it should be possible to use our synthetic RNA device as a general high-throughput screening platform for inconspicuous metabolite overproduction through accelerated evolution of microbes, thereby facilitating future efforts in metabolic engineering and synthetic biology [41] . 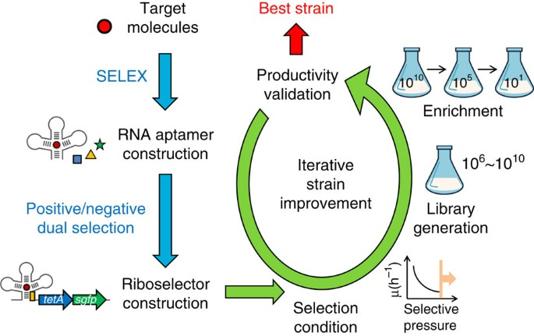Figure 4: Schematic diagram of iterative strain improvements driven by the Riboselector. RNA aptamer pools specific for target molecules are constructed by systematic evolution of ligand by exponential enrichment (SELEX). Using thesein vitro-selected aptamers, a Riboselector is generatedin vivothrough several rounds of dual positive and negative selection. After determining the selection condition for the parental strain using the Riboselector, the generated library can be enriched under the chosen selection pressure. Iterative strain improvement can be achieved by re-setting the selection conditions or re-constructing a Riboselector suitable for the newly developed parental strain. Figure 4: Schematic diagram of iterative strain improvements driven by the Riboselector. RNA aptamer pools specific for target molecules are constructed by systematic evolution of ligand by exponential enrichment (SELEX). Using these in vitro -selected aptamers, a Riboselector is generated in vivo through several rounds of dual positive and negative selection. After determining the selection condition for the parental strain using the Riboselector, the generated library can be enriched under the chosen selection pressure. Iterative strain improvement can be achieved by re-setting the selection conditions or re-constructing a Riboselector suitable for the newly developed parental strain. Full size image Bacterial strains and reagents The E. coli bacterial strains and plasmids used in this study are listed in Supplementary Table S3 . Oligonucleotides were synthesized by Bioneer (Daejeon, Korea) and are listed in Supplementary Table S4 . M9 media containing 4 g l −1 glucose, M9 salt solutions (Sigma, St Louis, MO, USA), 5 mM MgSO 4 , 0.1 mM CaCl 2 and appropriate antibiotics and supplements were used for cultivating each E. coli strain. Other reagents were obtained from Sigma (St Louis, MO, USA) unless otherwise indicated. Selection of the Tryptophan Riboselector An active Riboselector that specifically responds to L -tryptophan and regulates the expression level of downstream gene was selected by consecutive cycles of negative and positive selection. For negative selection, E. coli W3110 cells transformed with TrpRibo_Lib were collected, washed and inoculated at a final OD 600 of 0.05 into M9 medium containing 34 μg ml −1 chloramphenicol. After culturing for 12 h at 37 °C with shaking (200 rpm), the culture broth, inoculated to a final OD 600 of 0.005 into M9 medium containing 34 μg ml −1 chloramphenicol and 0.2 mM NiCl 2 , was incubated for 48 h. For positive selection, the cells that survived negative selection were collected, washed and inoculated at a final OD 600 of 0.05 into M9 medium containing 34 μg ml −1 chloramphenicol and 1 mM L -tryptophan. After culturing for 12 h at 37 °C with shaking (200 rpm), the culture broth was inoculated at a final OD 600 of 0.005 into M9 medium containing 34 μg ml −1 chloramphenicol, 1 mM L -tryptophan and 40 μg ml −1 tetracycline, and incubated for 24 h. After several rounds of negative and positive selection, the culture broth was streaked onto an Luria broth agar plate containing 34 μg ml −1 chloramphenicol, and incubated at 37 °C overnight to obtain isolated single colonies. The selected sequence of the random region used was 5′-GAGGGTAAGA-3′. When the selected plasmid was sequenced, there were two unexpected mutations in the aptamer region (Original sequence: 5′-ctggacgacggggacgccactggactaggtaagccaggaccgtacgtcgggagccgtcagaata-3′, selected sequence: 5′-ctggacgacggggacgccactggactaaggtaaccaggaccgtacgtcgggagccgtcagaata-3′). However, these mutations did not affect the function of the Tryptophan Riboselector, indicating that these mutations were either enriched to reflect the physiological condition or non-lethal to the function of riboswitch. The behaviour of Tryptophan Riboselector candidates was assessed by selecting several colonies and culturing them in M9 medium containing 34 μg ml −1 chloramphenicol with or without 1 mM L -tryptophan. After culturing for 12 h, fluorescence intensity was measured and normalized to the culture’s OD 600 value. The density of E. coli was measured at a wavelength of 600 nm using a UV-1700 spectrophotometer (Shimadzu, Kyoto, Japan). Fluorescence was detected using a VICTOR [3] 1420 Multilabel Counter (PerkinElmer, Waltham, MA, USA). The detection was carried out using a 486-nm excitation filter and a 535-nm emission filter with a 1-s measurement time. The activation ratio of the Tryptophan Riboselector was determined by dividing the normalized fluorescence of L -tryptophan-added broth by the normalized fluorescence of L -tryptophan-deficient broth. Implementation of the Riboselectors in metabolite producers Cellular growth rates as a function of intracellular metabolite concentration under the selection pressure were evaluated by culturing freshly prepared cells (WLN, WLM, WLR and WTR series) in 200 μl of M9 medium with appropriate antibiotics, supplements and selection pressures, namely NiCl 2 and tetracycline, and measuring the growth of each strain using BioscreenC MBR (Oy Growth Curves Ab, Helsinki, Finland). For survival tests in mixed culture, fresh culture broth of each strain, with or without Riboselectors, were inoculated at a final OD 600 of 0.025 each into M9 medium containing appropriate antibiotics, supplements and selection pressures (NiCl 2 for lysine strains and tetracycline for tryptophan strains). For comparisons of WLR2 and WLR3 strains, all amino acids except lysine were added to the medium to complement the metabolic burden of the WLR3 strain. After incubating for 12 h, the mixed culture broth was diluted in the same fresh medium and incubated for an additional 12 h. After four rounds of serial cultures, genomic DNA was extracted using an Exgene kit (GeneAll Biotechnology, Daejeon, Korea) and tested by PCR using primers corresponding to each strain (C-lysC-F and C-lysC-R2 for WLR1 and WLR2 mixed culture; C-iclR-F and C-iclR-R for WLR2 and WLR3 mixed culture; C-aroG-F and C-aroG-R for WTR0 and WTR1 mixed culture) to confirm that the relatively high-metabolite producers were enriched under the selection pressure. Enrichment experiments and population analysis of strains Growth inhibition of WLR3 and WLN3 strains was analysed by gradually changing the selection pressure (from 60 to 120 μM NiCl 2 ) to establish selection conditions under which the growth of WLR3 was stopped but that of WLN3 was not. The ppc promoter library (pCDF-ppc-Lib) was transformed into the either WLR4 or WLM4 and WLN4 (for control enrichments) strain, and cells were cultured in 30 ml of complemented M9 medium (supplemented with L -methionine and L -threonine to complement the auxotrophic phenotype of the WL3 strain) containing 90 μM NiCl 2 . After reaching an OD 600 value >0.6, cells were diluted in fresh selection medium. After three serial cultures (enrichment cycle 1), plasmids carrying the ppc promoter library were extracted and retransformed into fresh WLR4 or WLN4 cells to prevent the adaptation of cells to NiCl 2 . Enrichment cycles were performed four times and, after every cycle, plasmids were extracted from cells grown in enriched broth. Fragments containing the ppc promoter region were prepared by Bam HI restriction and analysed using a Genome Analyzer II (Illumina, San Diego, CA, USA). Lysine production and detection of metabolites The top three enriched strains (WLRE1, WLRE2 and WLRE3) using LysRibo, the parental strain (WL3), and three picked strains (WLNE1, WLNE2 and WLNE3) when used RiboNuLL, grown overnight in complemented M9 medium containing 40 μg ml −1 of streptomycin, were diluted to a final OD 600 of ~0.1 and cultured in the same medium until reaching an OD 600 of 0.8 (~8 h) to prepare fresh seeds. The culture broths were inoculated at a final OD 600 of ~0.05 into 15 ml of complemented M9 media in a 300-ml flask and incubated at 37 °C with shaking (200 rpm). The concentration of glucose consumed was determined by high-performance liquid chromatography (HPLC) with an Aminex HPX-87H column (Bio-Rad Laboratories, Richmond, CA, USA) at a flow rate of 0.6 ml min −1 at 65 °C using 5 mM H 2 SO 4 as the mobile phase. The glucose signal was monitored using a Shodex RI-101 detector (Shodex, Klokkerfaldet, Denmark). Lysine concentration in the broth was determined using a pre-column o-phthalaldehyde derivatization method [42] coupled with reversed-phase LC column chromatography (Acclaim 120 C18; Dionex, Sunnyvale, CA, USA) using an UltiMate 3000 analytical HPLC system (Dionex). Derivatized lysine was eluted at a flow rate of 1.5 ml min −1 with gradient of acetonitrile, methanol and water (v/v % 45:45:10) solution and 50 mM sodium acetate buffer (pH 6.5), and detected using a ultraviolet–vis diode array detector at 338 nm. Quantification of relative promoter strengths Promoter strengths of the enriched and parental strains were evaluated by first extracting total RNA from cells incubated for 6 h after inoculation using RNeasy Mini Kits and an RNase-free DNase system (Qiagen GmbH, Germany). cDNA preparation and real-time quantitative PCR were performed according to the manufacturer’s instructions. Relative ppc expression was quantified using the comparative C T method (ΔΔCt) using gapA as a reference [43] . How to cite this article: Yang, J. et al. Synthetic RNA devices to expedite the evolution of metabolite-producing microbes. Nat. Commun. 4:1413 doi: 10.1038/ncomms2404 (2013).